Reduced graphene oxide by chemical graphitization Reduced graphene oxides (RG-Os) have attracted considerable interest, given their potential applications in electronic and optoelectronic devices and circuits. However, very little is known regarding the chemically induced reduction method of graphene oxide (G-O) in both solution and gas phases, with the exception of the hydrazine-reducing agent, even though it is essential to use the vapour phase for the patterning of hydrophilic G-Os on prepatterned substrates and in situ reduction to hydrophobic RG-Os. In this paper, we report a novel reducing agent system (hydriodic acid with acetic acid (HI–AcOH)) that allows for an efficient, one-pot reduction of a solution-phased RG-O powder and vapour-phased RG-O (VRG-O) paper and thin film. The reducing agent system provided highly qualified RG-Os by mass production, resulting in highly conducting RG-O HI−AcOH . Moreover, VRG-O HI−AcOH paper and thin films were prepared at low temperatures (40 °C) and were found to be applicable to flexible devices. This one-pot method is expected to advance research on highly conducting graphene platelets. Recently, much attention has been paid to the production of large amounts of high-quality graphene platelets, which have attracted considerable attention for possible applications in various fields. Chemical graphitization from graphene oxide (G-O) to graphene has been introduced for mass production. The use of the vapour phase is needed to pattern hydrophilic G-Os on prepatterned substrates, as well as in in situ reduction to hydrophobic reduced graphene oxides (RG-Os). Moreover, a low-temperature process below the glass transition temperature is essential for flexible device fabrication on plastic substrates. Until now, the chemical reduction of G-O has entailed the use of hydrogen sulphide [1] , hydrazine [2] , NaBH 4 [3] , dimethylhydrazine [4] , hydroquinone [5] , the sequential use of NaBH 4 and H 2 SO 4 [6] , and aluminium powder [7] . Such reduction reagents have been reported to achieve a high degree of G-O reduction in the solution phase. Recently, electrochemical reduction methods have been introduced without the use of reducing reagents [8] , [9] . Until now, hydrazine hydrate, the most widely used reducing agent, was used in this work as a control to reduce G-O (RG-O NH2–NH2 ) in both the solution and gas phases. Unfortunately, the reducing agent gave rise to high sheet resistance because of the nitrogen impurities incorporated during the reduction process [10] . Therefore, a simple, one-pot process to restore the graphene structure is essential for obtaining high-quality RG-O for mass production. To realize the mass production of high-quality RG-O from G-O prepatterned on a plastic substrate, the development of new chemical reduction methods at low temperatures is needed in both gas and solution phases. Hydriodic acid with acetic acid (HI–AcOH) has been reported to efficiently convert polycyclic quinones and phenols into their corresponding arenes in excellent yield [11] . It was suggested that this organic reducing agent with iodide as a catalyst would replace the oxygen functional groups (epoxides and alcohols) with organohalides, which are good leaving groups, and produce high-quality RG-O in both solution and gas phases. It was also assumed that the reduction process would be possible even at room temperature, especially for a plastic substrate having low glass transition temperature, because of facile vapourization of HI into G-O. This paper reports the synthesis of high-quality RG-O through the HI–AcOH method using both solution and vapour phases for potential mass production. The highly efficient reduction of G-O powder and vapour-phased paper and thin film of prepatterned G-O onto a plastic substrate with HI–AcOH was examined systematically. We expect the conductivity of RG-O to increase dramatically in the powder, paper and thin film because of the high degree of deoxygenation and high graphitization without nitrogen incorporation. This novel approach may be used for the fabrication and processing of various RG-O papers and thin films in the development of new RG-O on flexible substrates, particularly for low temperature processes. RG-O powders Using solution and vapour phases with HI–AcOH, high-quality RG-O HI–AcOH suitable for mass production was prepared, as shown in Supplementary Figure S1 . A possible reduction mechanism is proposed in Supplementary Figure S2 [6] , [11] . The most informative analysis to support the reduction of G-O was elemental analysis (EA) of the raw graphite, G-O and RG-O ( Supplementary Table S1 ). The percentage of carbon in RG-O HI–AcOH was increased dramatically from 44.56 (G-O) to 82.63 (RG-O HI–AcOH ), whereas the percentage of oxygen decreased from 46.43 (G-O) to 7.21 (RG-O HI–AcOH ). The C/O ratios of RG-O HI–AcOH , highly RG-O [13] , chemically converted graphene (CCG) [14] and chemically converted graphene-2 (CCG2) [6] were 15.27, 11.0, 9.97 and 8.57, respectively, indicating the reduction to the largest extent of RG-O HI–AcOH among those of other RG-Os converted from G-Os. Furthermore, RG-O HI–AcOH did not contain any nitrogen atoms that would function as impurities in terms of the electrical conductance. As a result, reduction through HI provided higher levels of graphitization of graphene platelets compared with RG-Os produced using other reducing reagents. The dispersibility of the RG-O platelets showed a strong dependence on the degree of deoxygenation of the G-O platelets and their structure. In general, the G-O platelets could be well dispersed in water but not in dimethylformamide (DMF). On the other hand, after reducing the G-O platelets, the RG-Os could be easily dispersed in DMF. Similar to examples of dispersion of RG-O platelets carried out using other reductants and as described in the literature [15] , the RG-O HI–AcOH powder could be readily dispersed in DMF. The DMF dispersion was quite stable, showing no signs of agglomeration, even after 1 week. This is consistent with previous work, and is evidence of a high level of graphitization of the RG-O [15] . To estimate the stability of the RG-O HI–AcOH colloidal dispersion in various solvents when they are added to the existing DMF dispersion, 9 ml of various solvents, such as DMF, dimethylsulphoxide, N,N -dimethylacetamide, N -methylpyrrolidone, cyclohexanone, CH 3 CN, tetrahydrofuran, ethanol, toluene, o -dichlorobenzene and dichloromethane, were added to a DMF dispersion (0.3 mg RG-O HI–AcOH /1 ml DMF) and sonicated in a bath for 2 h, as shown in Supplementary Figure S3 . Polar solvents, such as dimethylsulphoxide, N,N -dimethylacetamide and N -methylpyrrolidone, produced stable homogeneous colloidal suspensions of RG-O sheets (at a 9:1 volume ratio of each to DMF). RG-Os HI–AcOH precipitated after several minutes to at most 1 day in nonpolar solvents, such as cyclohexanone, CH 3 CN, tetrahydrofuran, ethanol, toluene, o -dichlorobenzene and dichloromethane. Solvents with high polarity indices produced a stable dispersion of RG-O HI–AcOH , as summarized in Supplementary Table S2 . The colloidal hydrophobic nature of RG-O HI–AcOH in DMF ( ∼ 0.3 mg per 10 ml) was confirmed by the Tyndall light scattering effect, as shown in Supplementary Figure S4 [6] , [16] . Thermogravimetric analysis (TGA) was used to further assess the level of reduction of the G-O platelets. Fig. 1a displays the TGA thermograms that show weight loss as a function of temperature for dried-down G-O (at a heating rate of 1 °C min −1 ; higher heating rates can cause the material to rapidly expand and 'jump' out of the pan) and RG-O HI–AcOH (at a heating rate of 10 °C min −1 ) under a nitrogen atmosphere. The G-O sample showed significant weight loss with an onset temperature at slightly more than 100 °C, which was attributed to the elimination of interlamellar water, followed by loss of oxygen from the G-O platelets themselves (such as by evolution of CO and CO 2 from the sample) at slightly higher temperatures. RG-O HI–AcOH showed much higher thermal stability (weight loss of 12.05 wt% for RG-O HI–AcOH ) because of the better graphitization and deoxygenation of RG-O HI–AcOH with enhanced van der Waals forces between layers [17] , [18] , [19] . 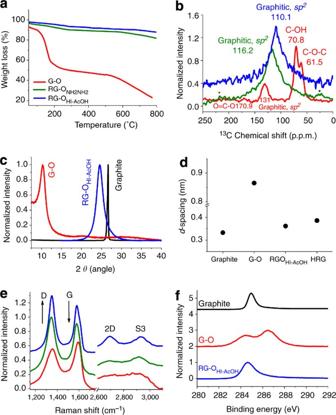Figure 1: Characterization of solution-phase RG-OHI−AcOHpowder. (a). Decomposition behaviour of G-O, RG-ONH2−NH2and RG-OHI−AcOH. (b)13C-MAS NMR spectra of G-O (red), RG-OHI−AcOH(blue) and RG-ONH2–NH2(green). * Indicates the spinning side bands20.(c) Powder XRD patterns of graphite, G-O and RG-OHI−AcOH. The 2θangles of the XRD peaks (d-spacing) of G-O and RG-OHI−AcOHshifted from 10.27° (d-spacing∼8.60 Å) to 24.57° (d-spacing∼3.62 Å) after reduction, respectively. (d)d-spacings for the indicated sample types. (e) Raman spectra of G-O (red), RG-OHI−AcOH(blue) and RG-ONH2–NH2(green). (f) XPS characterization indicates good restoration of graphite structures. Figure 1: Characterization of solution-phase RG-O HI−AcOH powder. ( a ). Decomposition behaviour of G-O, RG-O NH2−NH2 and RG-O HI−AcOH . ( b ) 13 C-MAS NMR spectra of G-O (red), RG-O HI−AcOH (blue) and RG-O NH2–NH2 (green). * Indicates the spinning side bands [20] . ( c ) Powder XRD patterns of graphite, G-O and RG-O HI−AcOH . The 2 θ angles of the XRD peaks ( d -spacing) of G-O and RG-O HI−AcOH shifted from 10.27° ( d -spacing ∼ 8.60 Å) to 24.57° ( d -spacing ∼ 3.62 Å) after reduction, respectively. ( d ) d -spacings for the indicated sample types. ( e ) Raman spectra of G-O (red), RG-O HI−AcOH (blue) and RG-O NH2–NH2 (green). ( f ) XPS characterization indicates good restoration of graphite structures. Full size image The 13 C magic angle spinning (MAS) NMR spectra ( Fig. 1b ) revealed a dramatic decrease in the oxygen functional groups for G-O at 170.9 (O=C–O), 70.8 (C–OH) and 61.5 (C–O–C) p.p.m., and new broad resonance peaks at 116.2 and 110.1 p.p.m. (graphitic, C sp 2 ) for RG-O NH2−NH2 and RG-O HI–AcOH , respectively, which is similar to the RG-Os reported in the literature [16] , [20] , [21] . The graphitic C sp 2 peaks of G-O (131.0), RG-O NH2−NH2 (116.2) and RG-O HI–AcOH (110.1 p.p.m.) were up-shifted and broadened and the more up-shifted C sp 2 peak of RG-O HI–AcOH compared with RG-O NH2–NH2 indicates that it is more graphite-like [6] , [16] . Sample spinning and probe tuning were found to be more difficult in the NMR measurement of the more electrically conducting RG-O HI−AcOH than for the RG-O NH2–NH2 and G-O samples. Ultimately, a 13 C NMR signal of RG-O HI–AcOH was obtained only at 200 MHz, as it could not be acquired at 400 or 600 MHz, even in a direct 13 C pulse experiment [6] . The powder X-ray diffraction (XRD) pattern of the prepared G-O was compared with those of the RG-Os depicted in Figure 1c . The peak position for graphite powder was 2 θ =26.7° ( d -spacing ∼ 3.34 Å). A typical broad peak near 10.27° ( d -spacing ∼ 8.60 Å) was observed for the G-O powder [22] . Compared with the parent G-O, the peak of RG-O HI–AcOH showed a dramatic shift to higher 2θ angles (24.57°; d -spacing ∼ 3.62 Å) and was narrower than that of highly RG-O ( ∼ 23°; d -spacing ∼ 3.86 Å) [12] , suggesting that RG-O HI–AcOH was well ordered with two-dimensional sheets without nitrogen incorporation and there was a decrease in the average interlayer spacing of the RG-O platelets depicted in Figure 1d . The thickness of the G-O platelet by atomic force microscopy (AFM) was similar to that reported in the literature, showing a height of approximately 1 nm [16] , as shown in Supplementary Figure S5 [12] . The RG-O HI–AcOH platelet on the SiO 2 substrate had a height of 0.66 nm (red line) and two overlapped layers had a height of 1.28 nm (blue line), as shown in Supplementary Figure S6 . The previously reported thicknesses for RG-O platelets measured in tapping AFM mode were 0.9–1.1 nm [23] for the sheet-to-substrate and 0.5-0.6 nm [14] for the sheet-to-sheet. Figure 1e presents the micro-Raman spectra of the graphitic layers in the powder samples. The peak for G-O (1594 cm −1 ) at the G-band was up-shifted compared with that of graphite (1580 cm −1 ) [24] . This was attributed to the presence of isolated double bonds that resonate at frequencies higher than that of the G-band of the graphite [25] . The G-band of RG-O HI–AcOH occurred at 1581 cm −1 , which corresponds to the recovery of the hexagonal network of carbon atoms with defects. The I D / I G ratio of RG-O HI–AcOH did increase notably, indicating that the reduction process altered the structure of G-O [26] with a high quantity of structural defects. The intensity of the two-dimensional ( ∼ 2680 cm −1 ) and S3 ( ∼ 2910 cm −1 ) peaks increased more than that of RG-O NH2–NH2 , showing better graphitization or no charge transfer due to the absence of nitrogen impurities in the RG-O NH2–NH2 [27] . Supplementary Figure S7 shows the X-ray photoemission spectroscopy (XPS) survey spectra of graphite, G-O and RG-O HI–AcOH powder samples. The C 1s and O 1s peaks were observed at 285 and 533 eV, respectively ( Supplementary Fig. S7 (a) ). Supplementary Figures S7 (b) and (c) show the C 1s spectra acquired from G-O and RG-O HI–AcOH samples, respectively. The XPS peaks of RG-O HI–AcOH at 285 eV in Figure 1f assigned to C are one main C–C and four small C–O components, which were observed in the C 1s peaks of the RG-O HI–AcOH : C–C (284.6 eV) for sp 2 carbon in graphite; C–O (286.5 eV); C=O (287.8 eV); C(O)O (289.1 eV) [21] . The peak intensities and atomic ratios (O 1s /C 1s ) of RG-O HI–AcOH in the C 1s peaks were decreased significantly in comparison with those of G-O. Table 1 lists the physical values of the powder XRD, Raman and XPS spectroscopy. Table 1 Spectroscopy of RG-O HI-AcOH powder. Full size table Figures 2a,c show transmission electron microscopy (TEM) images of the multilayered G-O and RG-O HI–AcOH platelets, respectively. Insets show magnified regions of the high-resolution TEM (HR-TEM) images. Selected area electron diffraction (SAED) was performed on this region along the [001] zone axis. The SAED patterns of G-O and RG-O HI−AcOH platelets were observed in the insets of Figures 2b,d , respectively. 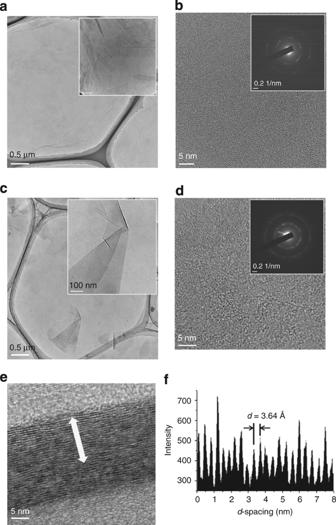Figure 2: TEM images of G-O and RG-OHI−AcOHplatelets. (a) and (c) HR-TEM images of stacks of G-O and RG-OHI−AcOHplatelets, respectively. The scale bar is 0.5 μm. Insets show magnified regions of the HR-TEM images. (b) and (d) SAED of stacks of G-O and RG-OHI−AcOHplatelets, respectively. (e) and (f) Cross-section of a stack of RG-OHI−AcOHplatelets. The diffraction pattern of the RG-O HI−AcOH platelets depicted in Figure 2d showed a crystalline structure. The first ring came from the (1100) plane and the bright spots corresponding to the (1100) reflections retained the hexagonal symmetry of the [0001] diffraction pattern [28] . The RG-O HI−AcOH platelets with more than six bright hexagonal spots might contain clustered defects arising from oxidation [29] . As these clusters were not fully restored into the hexagonal graphene framework, the RG-O HI−AcOH platelets have inclusions containing aperiodic decoration of functional groups [29] . Furthermore, the graphitic laminar structure of stacks of RG-O HI−AcOH platelets could be resolved in the 'ordered' region. Figure 2e shows a cross-section of one such stack and Figure 2f shows 22 layers in a ∼ 8 nm stack, the average interlayer distance of which was 3.64 Å, similar to that of the d -spacing (3.62 Å) obtained from XRD measurements (shown in Fig. 1c ). Fourier-transform infrared spectroscopy (FT-IR) spectra were recorded using a pressed disc of powder combined with KBr (1.0 mg powder per 200 mg KBr). Supplementary Figure S8 shows the FT-IR spectra of G-O and RG-O HI−AcOH . Oxygen functional groups of powder G-O showed stretching peaks at 1743 and 1624 cm −1 , and a broad band at 2431–3722 cm −1 . After reduction with HI–AcOH, the oxygen peaks decreased dramatically and the infrared transmission of RG-O HI−AcOH was decreased significantly compared with G-O, resulting in restoration of the electronic conjugation within the platelets, such as for electrically conducting carbon [30] . For the ultraviolet-visible (UV-vis) spectra of the G-O dispersion in DMF, the inset of Supplementary Figure S9 shows strong absorption bands at 293 and a shoulder peak at 360 nm: the maximum at 293 nm is from the π-plasmon of carbon [1] , and we assign the shoulder at 360 nm to the n →π* transitions of C=O. The UV-Vis spectra of G-O and RG-O HI−AcOH revealed RG-O HI−AcOH in DMF to have a relatively flat absorbance up to 900 nm, which is similar to that reported in the literature [14] , which corresponds to restoration of the electronic conjugation within the graphene sheets. Figure 2: TEM images of G-O and RG-O HI−AcOH platelets. ( a ) and ( c ) HR-TEM images of stacks of G-O and RG-O HI−AcOH platelets, respectively. The scale bar is 0.5 μm. Insets show magnified regions of the HR-TEM images. ( b ) and ( d ) SAED of stacks of G-O and RG-O HI−AcOH platelets, respectively. ( e ) and ( f ) Cross-section of a stack of RG-O HI−AcOH platelets. Full size image A standard halogen anion test was performed by combustion ion chromatography (CIC) connected to an automatic quick furnace (AQF-100) [31] , to determine the residual iodide (ionic forms of iodine) and iodate and iodine in the RG-O sample, which could conceivably affect the electrical conductivity. The detection limit of the CIC was 50 p.p.m. No iodo elements were found. For the electrical conductance measurements, RG-O pellets were prepared under an ∼ 15ton weight for 10 s using the KBr pellet method. The enhanced electrical conductivity resulted from better graphitization of C=C π-conjugation of the graphene basal plane and the decreased defects formed within the plane of RG-O HI−AcOH compared with the nitrogen-incorporated hydrazine system [18] . Table 2 and Supplementary Figure S10 summarize the electrical conductivity of the graphite and RG-O HI−AcOH powder pellets. The conductivity of the graphite and air-dried RG-O HI−AcOH powder pellets was 8.45 × 10 4 and 3.04×10 4 S m −1 , respectively, showing an almost fourfold increase with respect to the highest literature RG-O value (an air-dried CCG paper ∼ 7.2×10 3 S m −1 ) [14] . The high conductivity of the RG-O HI−AcOH was attributed to the lower structural defect density ( Table 2 ) [32] and closer restacking between the RG-O layers during the reduction process because of van der Waals forces. Table 2 Electrical properties of the RG-O HI–AcOH powder pellet and VRG-O HI–AcOH paper. 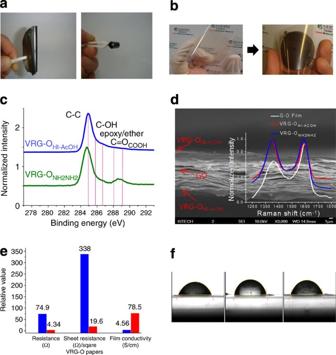Figure 3: Flexible VRG-OHI−AcOHpaper and thin film with G-O reduced in the gas phase. (a) Flexible VRG-OHI−AcOHpaper. (b) Flexible G-O (left) and VRG-OHI−AcOHthin films on a PET substrate. (c) XPS analysis of the C1sregion in VRG-OHI−AcOHand VRG-ONH2–NH2papers. A large loss of oxygen-functional groups after exposure to gas-phase reductants is evident. (d) SEM image of a cross-section and Raman spectra (inset) of VRG-OHI−AcOHpaper. (e) Electrical properties of VRGOHI−AcOH(blue) and VRG-ONH2–NH2(red) papers. VRG-OHI−AcOHpaper shows significantly higher electrical conductivity compared with the VRG-ONH2–NH2paper. (f) Water contact angles: (left) G-O (62.8°), (middle) VRG-OHI−AcOH(78.5°) and (right) VRG-ONH2–NH2(69.0°) papers. Full size table VRG-O papers Figure 3a , Supplementary Figure S11 and S12 provide detailed fabrication processes for the preparation of large-scale prepatterned G-O and vapour-phased RG-O (VRG-O) HI−AcOH paper (thickness ∼ 6.5 μm) and VRG-O NH2–NH2 , respectively, for possible applications of the conducting film to paper-like graphene. In XPS, the peak shape and position of the VRG-O HI−AcOH paper produced with HI were equivalent to those synthesized in the gas phase with hydrazine, with superior deoxygenation ( Fig. 3c and Supplementary Fig. S13 ). The SEM image of a cross-section of the VRG-O HI−AcOH paper in Figure 3d revealed a well-layered structure of the reduced G-O sheets. Raman spectroscopy, depicted in the inset of Figure 3d , shows that the increased I D / I G ratio of the RG-O HI−AcOH paper using the gas phase is analogous to that of RG-O HI−AcOH powder using both solution and gas phases, and this similarity suggests that the VRG-O HI−AcOH paper is essentially the same material as the RG-O HI−AcOH powder produced using both solution- and gas-phase reductants. Figure 3e shows the electrical properties of the flexibly fabricated VRG-O HI−AcOH ( Supplementary Fig. S11 ) and VRG-O NH2–NH2 ( Supplementary Fig. S12 ) [16] papers, and Table 2 summarizes their sheet resistances and conductivities. The sheet resistance and conductivity of the VRG-O HI−AcOH paper were 19.6 Ω square −1 and 7.85×10 3 S m −1 , respectively, which is more than 17 times higher than that of VRG-O NH2–NH2 (4.56×10 2 S m −1 ) prepared in this laboratory. Figure 3: Flexible VRG-O HI−AcOH paper and thin film with G-O reduced in the gas phase. ( a ) Flexible VRG-O HI−AcOH paper. ( b ) Flexible G-O (left) and VRG-O HI−AcOH thin films on a PET substrate. ( c ) XPS analysis of the C 1s region in VRG-O HI−AcOH and VRG-O NH2–NH2 papers. A large loss of oxygen-functional groups after exposure to gas-phase reductants is evident. ( d ) SEM image of a cross-section and Raman spectra (inset) of VRG-O HI−AcOH paper. ( e ) Electrical properties of VRGO HI−AcOH (blue) and VRG-O NH2–NH2 (red) papers. VRG-O HI−AcOH paper shows significantly higher electrical conductivity compared with the VRG-O NH2–NH2 paper. ( f ) Water contact angles: (left) G-O (62.8°), (middle) VRG-O HI−AcOH (78.5°) and (right) VRG-O NH2–NH2 (69.0°) papers. Full size image The surface morphology became rough as the reduction process progressed, as depicted in Supplementary Figure S14 . The level of reduction of the VRG-O HI−AcOH and VRG-O NH2–NH2 papers was further assessed by their wettability. Figure 3f shows the wettability of the G-O, VRG-O HI−AcOH and VRG-O NH2–NH2 papers. The water contact angles of the G-O, VRG-O HI−AcOH and VRG-O NH2–NH2 papers were 62.8°, 78.5° and 69.0°, respectively. The RG-O HI−AcOH surface had the highest hydrophobicity, providing the highest electrical conductance. VRG-O thin films on the plastic substrate The prepatterned G-O (left) depicted in Figure 3b was prepared on a polyethylene terephthalate (PET) substrate using a previously described vacuum filtration method [28] , followed by reduction to yield the VRG-O HI−AcOH (right) thin films. Conductivity of the VRG-O HI−AcOH thin film was approximately 9.44 S cm −1 , depending on film thickness ( d ∼ 100 nm). 13 C MAS NMR, XRD, HR-TEM and SAED analyses of RG-O powders clearly demonstrated that these HI–AcOH reduction methods can produce crystalline two-dimensional graphene platelets. No iodide ion or iodine molecules (as possible sources of electrical doping) were detected by combustion ion chromatography. The C/O ratio of the RG-O HI−AcOH platelets obtained from EA is one of the highest values and no nitrogen is present in the RG-O product material. This extensive reduction, along with a relatively small average interlayer distance as measured by both XRD and TEM (3.62 Å; 3.64 Å, respectively), is probably the main reason for the high electrical conductivity of paper-like samples composed of RG-O HI−AcOH platelets. In conclusion, this study examined a novel, one-pot chemical reduction method of G-O using HI–AcOH through the solution phase and prepatterned G-O through the gas phase. The conductivity of the RG-O increased dramatically in the powder, paper and thin film because of the high degree of deoxygenation and high graphitization without nitrogen incorporation. Furthermore, the simplicity of this method demonstrates the possibility of mass production through solution and gas phases and low-temperature processing with high conductivity on plastic substrates. This novel approach may be used for the fabrication and processing of various VRG-O papers and thin films in the development of new RG-O on flexible substrates, particularly for low-temperature processes. Chemicals and characterization Sulfuric acid (95–97%), hydrogen peroxide (30 wt%), potassium permanganate, sodium nitrate, hydriodic acid (57 wt%), hydrazine monohydrate (35 wt% in water, Aldrich), sodium bicarbonate and acetic acid were obtained from commercial sources and used as received. EA were performed on an LECO 932 Elementary Analyzer (Atlantic Microlab Inc). FT-IR spectra (KBr) were collected using a Thermo Nicolet AVATAR 320 instrument. All UV-vis absorption spectra were recorded using a double-beam UV-1650PC spectrophotometer (Shimadzu). 13 C MAS NMR spectra of G-O and RG-O NH2–NH2 samples were recorded on a spectrometer (Bruker Avance II-400) operating at a 10 kHz spinning rate for 13 C nuclei, applying the MAS technique. NMR spectroscopy of RG-O HI−AcOH was performed on a Varian 200 MHz solid-state NMR spectrometer equipped with a 4-mm probe at the Korea Basic Science Institute in Daegu Center, Korea. The direct 13 C-polarization spectrum was acquired with a 90° pulse of 3.5 μsec for a pulse repetition delay of 10 s for 8192 scans. The 13 C spectrum was referenced to TMS at 0 p.p.m. The thermal properties of the graphene platelets were characterized by TGA (Polymer Laboratories, TGA 1000 plus). All RG-O sample measurements were taken at a nitrogen gas flow rate of 40 ml min −1 over a temperature range of room temperature to 800 °C with a ramp rate of 10 °C min −1 . The G-O sample was also heated from room temperature to 800 °C at 1 °C min −1 to avoid thermal expansion of the G-O due to rapid heating. The exfoliated G-O and RG-O monolayers were characterized by AFM (Agilent Technologies, Agilent 5500 AFM/SPM System). Powder XRD patterns were recorded on a D8-Advance instrument (Germany) using Cu-Kα radiation. Raman spectroscopy measurements were taken using a micro-Raman system (Renishaw, RM1000-In Via) with excitation energy of 2.41 eV (514 nm). All XPS measurements were taken in a SIGMA PROBE (ThermoVG) using a monochromatic Al-Kα X-ray source at 100 W. Surface analyses of graphene papers were collected by optical microscopy (Microscopes Inc., wm0039000a S39A). The microstructure was observed by field emission scanning electron microscopy (JSM-6701F/INCA Energy, JEOL). HR-TEM imaging of G-O and RG-O HI−AcOH platelets and stacks of such platelets was performed on a JEOL JEM-2100F microscope at 200 keV. The TEM samples were prepared by dispersing dry powders of G-O and RG-O HI−AcOH in distilled water and methanol, respectively, to form a homogeneous suspension. The suspension was dropped on a 200 mesh copper TEM grid that was coated with a thin amorphous carbon film. SAED was performed in the TEM. To determine the possible residual iodide (ionic forms of iodine), and of iodate and iodine in the RG-O, a standard halogen anion test method was used with a CIC connected to an automatic quick furnace (AQF-100). The combustion apparatus (AQF-100, automatic quick furnace) was used for sample pretreatment. An ion chromatograph (Metrohm 761 compact IC) was used to determine the iodide and iodate and iodine content in the digested sample solutions following the combustion step. The certified halogen anion standards (each 1,000 p.p.m. solution) were obtained from Alltech. Distilled water was purified with a Milli-Q plus system (Millipore Co.) and the solutions were filtered through a 0.45 μm membrane filter and degassed. Oxygen and nitrogen were used for combustion at flow rates of 400 and 200 ml min −1 , respectively. Pyrolysis involved two steps. The first step increased the sample temperature in the shell oven to 700–900 °C. The second step increased the temperature of the sample to 800–1,000 °C with O 2 in the shell oven. This test was carried out on 0.10 g of RG-O and 30% H 2 O 2 absorption solution. An IonPac AS9-SC analytical column (Dionex), an IonPac AG9-SC guard column (Dionex) and a conductivity detector were used. The eluent consisted of a mixture of 1.8 mM Na 2 CO 3 and 1.7 mM NaHCO 3 . The flow rate was 1.5 ml min −1 and the injection volume was 100 μl. The diluted alkali absorption solution was then analysed by ion chromatography and the halogen element concentration of the absorption solution was determined using the standard curves. If the halogen element concentration of the absorption solution was above the calibration range, then it was diluted appropriately to a concentration within that range. The contact angles were measured using a SEO Phoenix 300 microscope at five different points. The conductivity was measured using a four-probe conductivity test metre (MCP-T600; Mitsubishi Chemical) at room temperature after pressing the samples into pellet or paper form. Preparation of G-O G-O was prepared from natural graphite powder (Bay Carbon, SP-1 graphite) using the modified Hummers and Offenman's method with H 2 SO 4 , NaNO 3 and KMnO 4 [12] , [33] . Preparation of RG-O HI−AcOH powder In a typical procedure, 4.0 g of G-O was dispersed in 1.5 l of acetic acid. This dispersion was sonicated using a Branson 1510 ultrasonic bath cleaner until it became clear. HI (80.0 ml) was then added and the mixture was stored at 40 °C for 40 h with constant stirring. The product was isolated by filtration, washed with saturated sodium bicarbonate (5×100 ml), distilled water (5×100 ml) and acetone (2×100 ml), and then vacuum dried overnight at room temperature to yield RG-O HI−AcOH (2.83 g) ( Supplementary Fig. S1 ). Preparation of RG-O NH2–NH2 powder The RG-O NH2–NH2 powder was reduced from G-O with hydrazine hydrate using the Wallace method [14] . Fabrication of G-O paper G-O powders were dispersed in D.I. water and the mixture was agitated homogeneously. Films were then prepared by solvent casting from the G-O solutions (10.0 ml) on clean glass Petri dishes (diameter, 5.0 cm). The water was evaporated slowly at room temperature for 2 days in a clean bench, followed by vacuum drying overnight at 50 °C, as shown in Supplementary Figure S12 (rectangle and circle shapes). Fabrication of VRG-O HI−AcOH paper The G-O paper was placed inside a 300 ml jar containing 2.0 ml of HI and 5.0 ml of acetic acid. The cover of the jar was sealed with vacuum grease and placed over an oil bath at 40 °C for 24 h. Subsequently, the VRG-O HI−AcOH papers were rinsed with a saturated sodium bicarbonate solution, water and methanol and dried at room temperature. The colour of the VRG-O HI−AcOH papers changed from matte brown to metallic grey after treatment with HI vapour, indicating the reduction of the materials, as depicted in Supplementary Fig. S11 . Fabrication of VRG-O NH2–NH2 paper The VRG-O NH2–NH2 paper was similarly prepared using a literature method [34] . Fabrication of VRG-O HI−AcOH thin films on plastic PET substrate The VRG-O HI−AcOH thin film was fabricated using a modification of a method reported elsewhere [15] . A dilute G-O suspension was vacuum filtered using a mixed cellulose ester membrane with 25 nm pores (Millipore). The G-O film was allowed to dry and adhere to the substrate at room temperature overnight under a 1.0 kg weight. The weight was removed and the membrane dissolved in acetone to leave the G-O thin film on the substrate. The G-O film was then rinsed with methanol and carefully transferred onto a PET film. The G-O/PET film was placed inside a 300 ml jar that contained 2.0 ml of HI and 5.0 ml of acetic acid. The cover of the jar was sealed with vacuum grease and placed in an oil bath at 40 °C for 24 h. Subsequently, the VRG-O HI−AcOH /PET film was rinsed with saturated sodium bicarbonate, water and methanol, and dried at room temperature. The colour of the VRG-O HI−AcOH /PET film changed from pale brown to pale black. How to cite this article: Moon, I.K. et al . Reduced graphene oxide by chemical graphitization. Nat. Commun. 1:73 doi: 10.1038/ncomms1067 (2010).